C(sp3)−C(sp3) bond formation via nickel-catalyzed deoxygenative homo-coupling of aldehydes/ketones mediated by hydrazine Aldehydes and ketones are widely found in biomass resources and play important roles in organic synthesis. However, the direct deoxygenative coupling of aldehydes or ketones to construct C(sp 3 )−C(sp 3 ) bond remains a scientific challenge. Here we report a nickel−catalyzed reductive homo-coupling of moisture- and air-stable hydrazones generated in-situ from naturally abundant aldehydes and ketones to construct challenging C(sp 3 )−C(sp 3 ) bond. This transformation has great functional group compatibility and can suit a broad substrate scope with innocuous H 2 O, N 2 and H 2 as the by-products. Furthermore, the application in several biological molecules and the transformation of PEEK model demonstrate the generality, practicability, and applicability of this novel methodology. The prospect of diminishing fossil hydrocarbon resources and the effects of global climate change call for the development of sustainable supply chains for the chemical industry that rely on renewable feedstocks [1] , [2] . Biomass, as a renewable resource, has the potential to provide earth rich and readily available carbon-based raw materials for chemical industry [3] . Although both biomass and fossil oil are carbon-based natural resources, their compositions are very different: while fossil feedstocks consist primarily of carbon and hydrogen, the oxygen content in biomass resources is very high mostly in the form of carbonyl or hydroxyl groups, which lead to complications and great challenges in the direct substitution of fossil resources with bio-based ones [4] , [5] , [6] . Therefore, the efficient transformation of these oxygen-containing compounds, especially the direct deoxygenation of aldehydes or ketones, could potentially provide an enabling tool for future biorefinery concepts. The formation of C(sp 3 )−C(sp 3 ) bond is one of the most fundamental strategies in organic transformations [7] , [8] , [9] . Especially, dibenzyl derivatives containing C(sp 3 )−C(sp 3 ) bond are essential structural motifs in natural products, pharmaceuticals and agrochemicals, as well as dyes and polymers [10] , [11] , [12] . Although the reductions of diarylalkenes and diarylalkynes provide means for the preparation of bibenzyl compounds [13] , [14] , homo-coupling strategies show superiority to access these compounds. For example, the homo-coupling of benzyl halides [15] , benzylmagnesium halides [16] , phenylacetic acids [17] , benzyl boronic acids [18] and methylbenzene derivatives [19] have been disclosed in recent years. However, these methods suffered from several drawbacks such as the tedious prefunctionalization steps, the use of moisture-sensitive organometallic reagents and the requirement of noble metals, which greatly limit their broad applicability. Therefore, the development of a novel approach for the direct formation of C(sp 3 )−C(sp 3 ) bond from naturally abundant aldehydes/ketones would be highly desirable. The Wolff–Kishner reduction is a classical direct deoxygenation strategy for converting aldehydes/ketones into alkane derivatives mediated by hydrazine (Fig. 1a ) [20] . Inspired by this classical reaction, great progress toward C–C bond construction using simple hydrazones, readily generated in situ from aldehydes/ketones and hydrazine, as nucleophiles through deoxygenative cross-coupling strategies have been made by us [21] , [22] , [23] , [24] , [25] , [26] , [27] and others [28] , [29] , [30] over the past several years. Moreover, as a strong reductant, hydrazine itself was also successfully applied as a reductant in reductive coupling reactions with aryl halides [31] . Inspired by the transformation of Wolff–Kishner reduction and our previous work [21] , [31] , we turned to consider whether hydrazine can also serve as a reductant for the reductive coupling of carbonyls to realize C(sp 3 )−C(sp 3 ) bond formation. Fig. 1: Strategies for deoxygenation of aldehydes and ketones with hydrazine. a Wolff–Kishner reductive deoxygenation of aldehydes (ketones). b Nickel-catalyzed deoxygenative homocoupling of aldehydes (ketones). Full size image Here, we show a powerful and reliable strategy in which nickel-catalyzed the direct deoxygenative homo-coupling of aldehydes/ketones mediated by hydrazine to synthesize dibenzyl derivatives (Fig. 1b ). Highlighted features of this protocol are: (a) H 2 O, N 2 and H 2 as innocuous side products; (b) naturally rich aldehydes/ketones as homo-coupling materials; (c) overcome the competing Wolff–Kishner reaction in the presence of base; (d) inexpensive and earth-abundant nickel as catalyst; (e) broad substrate scope and great functional group tolerance; and (f) synthesis of commercial drug molecule and transformation of PEEK model. 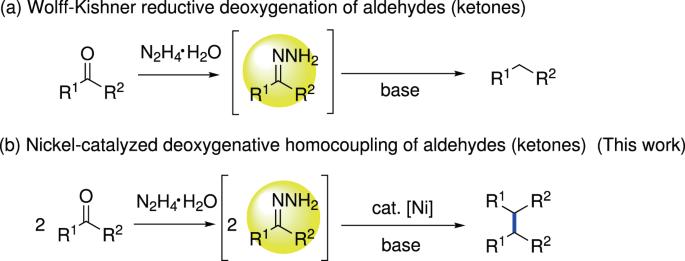Fig. 1: Strategies for deoxygenation of aldehydes and ketones with hydrazine. aWolff–Kishner reductive deoxygenation of aldehydes (ketones).bNickel-catalyzed deoxygenative homocoupling of aldehydes (ketones). Reaction optimization To initiate the exploration, hydrazone 2a generated from benzaldehyde ( 1a ) was chosen as the model substrate to optimize the reaction conditions (Table 1 ). The deoxygenative homo-coupling product 3a was obtained in 30% yield when NiCl 2 (20 mol%) was used as catalyst in presence of trimethylphosphine (PMe 3 , 40 mol%), using 1,8-diazabicyclo[5.4.0]undec-7-ene (DBU) as base and THF as solvent under an argon atmosphere at 100 °C for 24 h (Table 1 , entry 1). Other nickel catalysts, such as NiBr 2 , Ni(acac) 2 ∙4H 2 O, Ni(OAc) 2 , NiCl 2 (PPh 3 ) 2 and Ni(cod) 2 , also gave the desired products, but showed relatively lower efficiency (Table 1 , entries 2–6). Notably, in absence of any key component, including catalyst, ligand or base, no desired product 3a was obtained (Table 1 , entries 7–9). According to our previous work [26] , [27] , base plays a key role in the hydrazone conversion process, and the strong base is more favorable than the weak one. Therefore, other bases were examined: organic bases including DABCO and Et 3 N showed lower efficiency than DBU (Table 1 , entries 10–11), which is consistent with the previous work; inorganic bases such as KOH and t-BuOK may have poor solubility in the catalytic system, making the reaction yield markedly reduced (Table 1 , entries 12–13). In addition to the monodentate phosphine ligand, other phosphorus, nitrogen and carbene ligands were also tested, with N-heterocyclic carbene in situ generated from 1,3-bis(2,4,6-trimethylphenyl)imidazolium chloride (IMes∙HCl) giving the best result (Table 1 , entries 14–23). To our satisfaction, the reaction yield reached 65% when using 1,4-dioxane instead of THF as the solvent (Table 1 , entry 24). Based on this, when the amount of catalyst and ligand were increased to 30 mol%, 83% yield of 3a could be obtained (Table 1 , entry 25). Finally, the effect of temperature on the reaction was also investigated (Table 1 , entries 26–27). When the temperature was decreased to 80 °C, the starting material hydrazone could not be completely converted, indicating that the reaction rate is insufficient at low temperature. Due to the detection of a large amount of Wolff–Kishner reduction by-product at 120 °C, the yield of homo-coupling product decreased significantly. 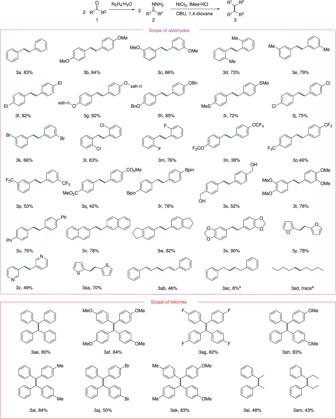Fig. 2: Substrate scope of the homo-coupling reaction. General conditions:2(2 × 0.1 mmol), NiCl2(0.03 mmol, 30 mol%), IMes∙HCl (0.03 mmol, 30 mol%), DBU (0.22 mmol, 2.2 equiv) and 1,4-dioxane (1.0 mL) at 100 °C for 24 h under an argon atmosphere, isolated yields.aDetected by GC-MS. Table 1 Optimization of the reaction conditions a . Full size table Investigation of the substrate scope To assess the generality of this method, the scope of the nickel-catalyzed deoxygenative homo-coupling process was examined, as shown in Fig. 2 . In general, this reaction demonstrated good functional group tolerance with respect to the substitution patterns and electronic properties of hydrazones generated from aldehydes. A variety of aryl aldehydes bearing electron-donating groups (methoxy-, methyl-, ethyl-, alkoxy- and methylthio-) or electron-withdrawing groups (halogen-, trifluoromethoxy- trifluoromethyl- and ester-) at different positions (ortho-, meta- or para-) of the aryl ring were smoothly converted to the homo-coupling products in moderate to excellent yields ( 3b-3q ). It was noteworthy that the hydrazone bearing a borate group was able to deliver the corresponding dibenzyl boronic esters 3r , which provides a handle for downstream transformations. Furthermore, the substrate bearing an unprotected hydroxymethyl group gave the product 3s . In addition, the multisubstituted substrate could be tolerated in this catalytic system, affording the desired product 3t . To our gratification, various polycyclic (hetero-) aromatic structures such as biphenyl, naphthalene, indene, dioxole, furan, pyridine and thiophene on aldehydes could also be tolerated in the transformation with moderate to good yields ( 3u - 3aa ). Because 1,5-dienes are valuable building blocks in organic synthesis and medicinal chemistry [32] , the desired 1,5-diene product 3ab was successfully synthesized through this nickel-catalyzed system using cinnamaldehyde-derived hydrazone as a substrate. Unfortunately, for valeraldehyde and phenylacetaldehyde substrates, only 8% or trace yield of the desired products ( 3ac - 3ad ) was detected by GC-MS, probably due to the competing azine formation under high temperature. Fig. 2: Substrate scope of the homo-coupling reaction. General conditions: 2 (2 × 0.1 mmol), NiCl 2 (0.03 mmol, 30 mol%), IMes∙HCl (0.03 mmol, 30 mol%), DBU (0.22 mmol, 2.2 equiv) and 1,4-dioxane (1.0 mL) at 100 °C for 24 h under an argon atmosphere, isolated yields. a Detected by GC-MS. Full size image Subsequently, the scope of hydrazones generated from ketones was investigated (Fig. 2 ). Symmetric diaryl ketones bearing various substituents were suitable substrates, providing the corresponding products 3ae - 3ag in excellent yields. To our delight, the homo-coupling reaction also occurred smoothly with non-symmetrical diaryl ketones as substrates, afforded the dibenzyl products ( 3ah - 3aj ) in 46–84% yields. In particular, the non-symmetrical diphenyl ketone (4-methoxyphenyl)( p -tolyl)methanone, which contains different substituents, gave the homo-coupling product 3ak . Moreover, aryl alkyl ketone, such as acetophenone and propiophenone, were all suitable substrates for this transformation, providing moderate yields of the desired products 3al - 3am . Applications To further exploit the practicality of current protocol, a gram-scale experiment of 2a generated from benzaldehyde ( 1a ) was conducted, and the product 3a was obtained in 75% yield (1.09 g) after 36 h (Fig. 3a ). In addition, to evaluate its synthetic applications, the drug molecule Britonin A ( 6 ) was synthesized from naturally abundant 4 under standard reaction conditions (Fig. 3b ). Polyetheretherketone (PEEK), being one of the most commonly used engineering plastics in industry, has caused waste accumulation problems due to its stability [33] . Therefore, the conversion of disused PEEK into other useful chemicals is a sustainability challenge. To our delight, when the PEEK model compound 7 (Fig. 3c ) was tested with this nickel-catalyzed system, the desired homo-coupling product 9 was obtained in 67% yield, which was confirmed by X-ray analysis (see the Supplementary Information ). These results indicated that the utility of our protocol for the late stage synthesis and modification of complex molecules. Fig. 3: Applications of the deoxygenative aldehyde/ketone homo-coupling. a Gram-scale experiment. b Synthesis of Britonin A. c Conversion of polyetheretherketone (PEEK) model compound. Full size image Mechanistic studies In order to gain mechanistic insights, some preliminary experiments were subsequently carried out. Firstly, the efficiency of the model reaction was almost unaffected in the presence of free radical initiator 2,2,6,6-tetramethyl-1-piperidinyloxy (TEMPO), demonstrating an unlikely radical pathway in this transformation (Fig. 4a ). Secondly, deuterium-labeling experiment using deuterated hydrazone d-2a was performed under standard conditions, and the homo-coupling product d-3a was obtained in 72% yield with 80% deuteration at benzylic position, which attributed the origination of hydrogen at the benzylic position to the N–H group in hydrazone (Fig. 4b ). Thirdly, dibenzalhydrazine ( 10 ), which appeared at a trace amount in the reaction, was prepared and examined under the standard conditions, and no desired product 3a was detected, demonstrating the improbable process involving azine as a reaction intermediate (Fig. 4c ). Finally, when ( E )−1,2-diphenylethene ( 11 ) was tested, only a small amount of the corresponding product 3a was obtained in the presence of hydrazine (Fig. 4d ) or hydrazone 2b (Fig. 4e ), indicating that the ( E )−1,2-diphenylethene is unlikely an intermediate in this deoxygenative homo-coupling process either. Fig. 4: Mechanistic studies. a Free radical capture experiment. b Deuterium-labeling experiment. c Experiment to verify possible azine intermediate. d Experiment to verify possible intermediate ( E )−1,2-diphenylethene reacting with hydrazine. e Experiment to verify possible intermediate ( E )−1,2-diphenylethene reacting with hydrazone 2b . Full size image Based on the above experimental results and our previously reported works [34] , [35] , we proposed a plausible reaction mechanism, as depicted in Fig. 5 . Initially, the active nickel (II) species A potentially coordinates with hydrazone anion to form nickel (II) complex B , which rapidly releases N 2 gas through Wolff−Kishner reaction-like process and an intramolecular benzyl migration to obtain intermediate C [35] . Next, intermediate C combines with another hydrazone anion to form the intermediate E via the nickel (II) complex D . Finally, reductive elimination and hydrogen generation provides the desired homo-coupling product 3 and regenerates the active catalyst. It is also possible to combine the active nickel species A with two molecules of hydrazone anions, followed by intramolecular migration, deprotonation and release of N 2 to obtain the desired product. More explorations of mechanistic details of this protocol are undergoing in our laboratory. Fig. 5: Proposed mechanism. Possible reaction mechanism of deoxygenative homo-coupling of aldehydes/ ketones. L n means ligand. Full size image In conclusion, a direct deoxygenative homo-coupling of hydrazones generated in situ from naturally abundant aldehydes or ketones to construct C(sp 3 )−C(sp 3 ) bond has been established, catalyzed by earth-abundant nickel. 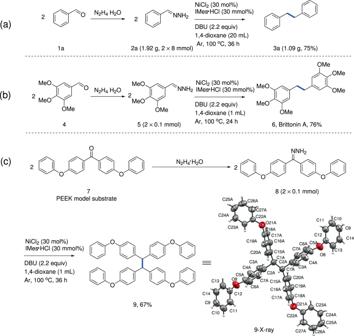Fig. 3: Applications of the deoxygenative aldehyde/ketone homo-coupling. aGram-scale experiment.bSynthesis of Britonin A.cConversion of polyetheretherketone (PEEK) model compound. This protocol is under mild reaction conditions with a broad substrate scope bearing a wide range of functional groups. Furthermore, this homo-coupling protocol can be applied to the rapid synthesis of some complex molecules such as Brittonin A and the transformation of PEEK model substrates. Most importantly, this hydrazine-mediated homogeneous catalytic process enables the preparation of high value-added bibenzyl derivatives from simple and readily available raw materials and provides a useful alternative for C(sp 3 )−C(sp 3 ) bond formation. General procedure for reactions in Table 1 A flame-dried V-shape reaction vial (10 cm 3 ) equipped with a magnetic stir bar was transferred into the glovebox and was charged with catalyst, ligand, and base, hydrazones (2 × 0.1 mmol) and solvent (1 mL). Then, the reaction vessel was sealed, moved out of the glovebox, and placed in a preheated oil bath. The mixture was stirred under an argon atmosphere. After completion of the reaction, the reaction mixture was cooled to room temperature and concentrated, and then dibromomethane (7 µL, 0.1 mmol) was added into the mixture as standard. The crude mixture was diluted by CDCl 3 to run the 1 H NMR test to determine the 1 H NMR yield. 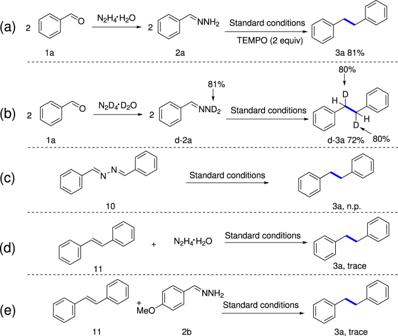Fig. 4: Mechanistic studies. aFree radical capture experiment.bDeuterium-labeling experiment.cExperiment to verify possible azine intermediate.dExperiment to verify possible intermediate (E)−1,2-diphenylethene reacting with hydrazine.eExperiment to verify possible intermediate (E)−1,2-diphenylethene reacting with hydrazone2b. 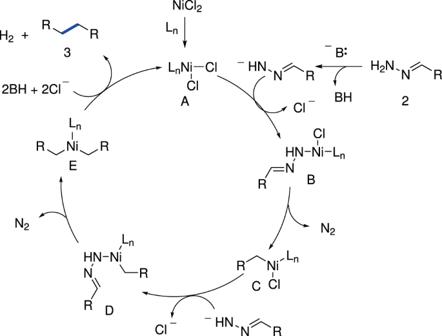Fig. 5: Proposed mechanism. Possible reaction mechanism of deoxygenative homo-coupling of aldehydes/ ketones. Lnmeans ligand. General procedure for reactions in Figs. 2 , 3 and 4 A flame-dried V-shape reaction vial (10 cm 3 ) equipped with a magnetic stir bar was charged with NiCl 2 (3.9 mg, 30 mol%), IMes∙HCl (10.2 mg, 30 mol%) and hydrazones (2 × 0.1 mmol). The vial was transferred into the glovebox and charged with 1,4-dioxane (1 mL) and DBU (33 µL, 0.22 mmol) before being sealed with a rubber septum. The tube was placed in a preheated oil bath at 100 °C and the mixture was stirred under an argon atmosphere for 24–36 h. The reaction mixture was cooled to room temperature and concentrated, and then was purified by preparative TLC on silica gel eluting with hexane: EtOAc (50:1-2:1) to afford the products. (Note: For Figs. 4 a, 2 equiv of TEMPO were added into the reaction; for Fig. 4b , replace hydrazone with deuterated hydrazine; for Fig. 4c , replace hydrazone with dibenzalhydrazine; for Fig. 4d , replace hydrazone with ( E )−1,2-diphenylethene and added N 2 H∙H 2 O (0.2 mmol); for Fig. 4e , replace hydrazone with ( E )−1,2-diphenylethene and added hydrazone 2b (0.2 mmol)).